Anoctamin 6 mediates effects essential for innate immunity downstream of P2X7receptors in macrophages Purinergic P2X 7 receptors (P2X 7 R) are fundamental to innate immune response. In macrophages, transient stimulation of P2X 7 R activates several transport mechanisms and induces the scrambling of phospholipids with subsequent membrane blebbing and apoptosis. These processes support phagocytosis and subsequent killing of phagocytosed bacteria. Here we demonstrate that the stimulation of P2X 7 receptors activates anoctamin 6 (ANO6, TMEM16F), a protein that functions as Ca 2+ dependent phospholipid scramblase and Ca 2+ -activated Cl − channel. Inhibition or knockdown of ANO6 attenuates ATP-induced cell shrinkage, cell migration and phospholipid scrambling. In mouse macrophages, Ano6 produces large ion currents by stimulation of P2X 7 receptors and contributes to ATP-induced membrane blebbing and apoptosis, which is largely reduced in macrophages from Ano6 −/− mice. ANO6 supports bacterial phagocytosis and killing by mouse and human THP-1 macrophages. Our data demonstrate that anoctamin 6 is an essential component of the immune defense by macrophages. P2X 7 receptors (P2X 7 R) are ligand-gated non-selective cation channels that are activated by high concentrations of extracellular nucleotides, which may be released during inflammation, tissue injury and T-cell activation [1] , [2] . P2X 7 R has a unique large C terminus, which may couple to multiple intracellular signalling pathways [3] , [4] . Activation of P2X 7 R not only leads to an instantaneous inward cationic current, but also to the formation of a non-selective pore, permeable to molecules up to 900 Da, which eventually leads to cell lysis [5] , [6] . In fact, distinct pores for P2X 7 R-activated uptake of cationic and anionic fluorescent dyes have been proposed [7] , [8] , while a contribution of the hemichannel pannexin 1 is discussed controversially [3] , [9] , [10] , [11] , [12] , [13] . It remains currently unclear whether the concept of pore dilation of P2X 7 R (ref. 14 ) is sufficient to explain the large conductance associated with P2X 7 R, and to what extend other ion channels may contribute. ANO6 (anoctamin 6, TMEM16F) is a Ca 2+ -dependent phospholipid scramblase [15] , [16] , [17] and a putative Ca 2+ -activated Cl − and non-selective cation channel [18] , [19] , [20] , [21] that is activated during apoptotic cell death [22] , [23] , [24] . ANO6 facilitates apoptotic cell shrinkage and is a component of the ubiquitous outwardly rectifying Cl − channel that has been identified in many cell types [22] , [24] . This scramblase/channel is activated by high intracellular Ca 2+ concentrations, as they occur during activation of P2X 7 (refs 14 , 15 , 25 ). We therefore asked whether the stimulation of P2X 7 R activates ANO6, and whether both Ca 2+ and the large C terminus of P2X 7 contribute to activation of ANO6. P2X 7 receptors show highest expression in macrophages, where they are important for innate immunity during infectious diseases [26] , [27] , while ANO6 was found to be expressed in spleen, osteoclasts and immune cells [15] , [17] , [22] , [28] , suggesting an overlapping expression. A cascade of cellular events is triggered through the stimulation of P2X 7 R, with the initial activation of non-selective cation currents and a subsequent pore conductance. This is followed by sequential cell shrinkage/swelling, phospholipid scrambling, membrane blebbing and finally cell death [2] , [29] , [30] , [31] . The aim of the present study was, therefore, to examine whether ANO6 and P2X 7 R are coexpressed in macrophages and whether ANO6 mediates some of the cellular effects downstream of P2X 7 R. These questions were tackled by analysing the activation of ANO6 through stimulation of P2X 7 R in overexpressing Xenopus oocytes and HEK293 cells, and in human and mouse macrophages from wild-type (wt) and Ano6 -knockout mice. P2X 7 R activates a large conductance in Xenopus oocytes Pore formation by stimulation of P2X 7 R expressed in Xenopus oocytes has been proposed earlier [32] . We expressed hP2X 7 R in Xenopus oocytes and observed very large delayed activated currents on continuous stimulation by 1 mM ATP ( Fig. 1a,b ). These pore currents were not observed in water-injected oocytes, and were not due to activation of endogenous Ca 2+ activated Cl − currents (xAno1), since whole-cell currents activated by the Ca 2+ ionophore ionomycin were negligible when compared with P2X 7 R pore currents ( Fig. 1c , Supplementary Fig. 1a ). Activation of large currents was inhibited by blockers of P2X 7 R, such as HMA (5-( N , N -hexamethylene)-amiloride) and AZ11645373 ( Supplementary Fig. 1b ). Xenopus oocytes express endogenous xAno6, as demonstrated by reverse transcription-PCR (RT–PCR; Fig. 1d ). Because a substantial portion of delayed P2X 7 R-activated currents was inhibited by blockers of Ano6, like niflumic acid (NFA), NPPB (5-nitro-2-(3-phenylpropylamino) benzoic acid) and tannic acid (TA) [33] , a contribution of xAno6 to the large current was suggested ( Fig. 1f ). Notably, NFA blocked the activation of a large pore current in Xenopus oocytes also in a previous study [34] . The inhibitors had no significant effects on immediate P2X 7 R currents activated within 1 s of ATP application but blocked delayed (after 3 min) currents, suggesting inhibition of xAno6 but not a direct inhibition of P2X 7 R by these blockers ( Fig. 1e,f ). Moreover, we injected sense or antisense DNA for xAno6 into ooyctes 3 days before injecting cRNA for P2X 7 R, and 6 days before performing the DEVC experiments. We found that the whole-cell current activated by ATP was significantly reduced by about 45% in oocytes injected with antisense DNA ( n =28), when compared with oocytes injected with sense DNA ( n =30; Supplementary Fig. 1c ). 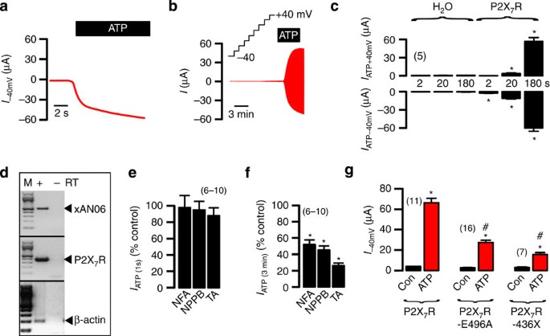Figure 1: Stimulation of P2X7R activates a pore current inXenopusoocytes that is inhibited by inhibitors of Ano6. (a) Whole-cell currents (holding voltage =−40 mV) activated by 1 mM ATP in aXenopusoocyte expressing P2X7R. (b) Continuous recording of whole-cell currents (clamp voltage ±40 mV in steps of 10 mV) activated by ATP in a P2X7R-expressing oocyte. (c) Summary of whole-cell currents in water-injected control or P2X7R-expressing oocytes measured 2, 20 and 180 s, respectively, after the application of ATP. (d) RT–PCR analysis of endogenousxAno6, overexpressed P2X7R, and β-actin. M=marker, ±reverse transcriptase (RT). (e,f) Inhibition of whole-cell currents (%) by NFA (10 μM), 5-nitro-2-(3-phenylpropylamino) benzoic acid (NPPB; 100 μM) and TA (20 μM), when measured 1 s (e) or 3 min (f) after application of ATP. (g) Summary of whole-cell currents before and after stimulation with ATP of oocytes expressing P2X7R (wt), P2X7R-E496A and P2X7R-436X, respectively. All currents were measured using double electrode voltage-clamp techniques. Mean±s.e.m.,n=number of cells.#significant difference to P2X7R (P<0.05; analysis of variance). *significant activation by ATP or inhibition by channel blockers (P<0.05; pairedt-test). Figure 1: Stimulation of P2X 7 R activates a pore current in Xenopus oocytes that is inhibited by inhibitors of Ano6. ( a ) Whole-cell currents (holding voltage =−40 mV) activated by 1 mM ATP in a Xenopus oocyte expressing P2X 7 R. ( b ) Continuous recording of whole-cell currents (clamp voltage ±40 mV in steps of 10 mV) activated by ATP in a P2X 7 R-expressing oocyte. ( c ) Summary of whole-cell currents in water-injected control or P2X 7 R-expressing oocytes measured 2, 20 and 180 s, respectively, after the application of ATP. ( d ) RT–PCR analysis of endogenous x Ano6, overexpressed P2X 7 R, and β-actin. M=marker, ±reverse transcriptase (RT). ( e , f ) Inhibition of whole-cell currents (%) by NFA (10 μM), 5-nitro-2-(3-phenylpropylamino) benzoic acid (NPPB; 100 μM) and TA (20 μM), when measured 1 s ( e ) or 3 min ( f ) after application of ATP. ( g ) Summary of whole-cell currents before and after stimulation with ATP of oocytes expressing P2X 7 R (wt), P2X 7 R-E496A and P2X 7 R-436X, respectively. All currents were measured using double electrode voltage-clamp techniques. Mean±s.e.m., n =number of cells. # significant difference to P2X 7 R ( P <0.05; analysis of variance). *significant activation by ATP or inhibition by channel blockers ( P <0.05; paired t -test). Full size image Activation of currents was largely reduced, but not completely inhibited, by the removal of extracellular Ca 2+ , suggesting Ca 2+ -dependent- and Ca 2+ -independent components of the large whole-cell conductance [8] ( Supplementary Fig. 1d ). In contrast, chelation of intracellular Ca 2+ by preincubation of the oocytes with 1,2-Bis(2-amino-5-methylphenoxy)ethane- N , N , N ′, N ′-tetraacetic acid tetrakis(acetoxymethyl) ester (BAPTA-AM; 0.1–1 mM) had no effects on activation of currents ( Supplementary Fig. 1d ). The current was also attenuated by mutating (hP2X 7 R-E496A) or truncating (hP2X 7 R-436X) the C terminus of P2X 7 R, suggesting requirement of both Ca 2+ influx and the C terminus of P2X 7 R for activation of the large currents ( Fig. 1g ). Notably, the removal of extracellular Cl − inhibited the inward current rather than the outward current, a phenomenon that was observed earlier for P2X 7 R expressed in HEK293 cells [35] . However, replacement of extracellular Na + by NMDG + only partially inhibited ATP-activated whole-cell currents, suggesting a permeability for large cations like NMDG + , as observed earlier [32] ( Supplementary Fig. 1e ). P2X 7 receptors and Ca 2+ activate ANO6 currents When expressed in HEK293 cells, ANO6 localized to the cell membrane and produced a whole-cell current at high intracellular Ca 2+ concentrations, or when stimulated with the Ca 2+ ionophore ionomycin ( Supplementary Fig. 2a–c ). Some currents were also activated in mock-transfected cells probably due to the activation of endogenous ANO6 ( Supplementary Fig. 2b ) [18] . ANO6 whole-cell currents remained outwardly rectifying in an extracellular Na + -free bath solution, but changed from outwardly rectifying to more linear currents when Na + was present in the bath solution, suggesting delayed activation of non-selective ANO6 currents ( Supplementary Fig. 2d ) [19] . ANO6 currents were partially inhibited by Cl − removal and were blocked by NFA, DIDS (4,4'-diidothiocyano-2,2'-stilbenedisulphonic acid), NPPB and TA ( Supplementary Fig. 2e ). The current exhibited an Eisenman type 1 anion selectivity sequence ( Supplementary Fig. 2f ) [19] . In HEK293 cells overexpressing P2X 7 R, high extracellular ATP (3 mM) activated an immediate inward current that was followed by a somewhat delayed more linear current [14] ( Fig. 2a ). No currents were activated in the absence of P2X 7 R ( Fig. 2b ). Linear currents were significantly reduced by the knockdown of ANO6, using two different short interfering RNAs (siRNAs; Fig. 2a,b , Supplementary Fig. 3a ). ANO6 knockdown was also verified by real-time RT–PCR, which indicated a knockdown by 76.4±3.7% (siRNA1; n =3) and 66.5±1.7% (siRNA2; n =3). The immediate P2X 7 R inward current was not affected by siRNA-ANO6, suggesting that the observed whole-cell current is the sum of P2X7 and ANO6 currents ( Fig. 2a ). Although our experiments cannot definitely separate between pure P2X 7 R currents and Ca 2+ activated ANO6 currents, we found that the ANO6 blocker TA inhibited delayed activated currents (3 min after application of ATP), but not instantaneous currents (1 s after ATP; Fig. 2d , Supplementary Fig. 4a ). Moreover, the coexpression of P2X 7 R and ANO6 further augmented ATP-activated currents, while the coexpression of ANO6 with P2X 7 R-E496A showed reduced current activation ( Fig. 2b,c ). No currents were activated by ATP in the absence of P2X 7 R. Fura-2-measurements indicated a strong and sustained increase in intracellular [Ca 2+ ] by ATP in P2X 7 R-expressing cells ( Fig. 2e,f ). These experiments demonstrate the activation of ANO6 by P2X 7 R in HEK293 cells. Together with the results obtained in Xenopus oocytes ( Fig. 1g ), we may suggest a role of the P2X 7 R C terminus for current activation [36] . Evidence for a possible direct interaction of P2X 7 R with ANO6 was detected by coimmunoprecipitation of both proteins overexpressed in HEK293 cells ( Supplementary Fig. 4b ). 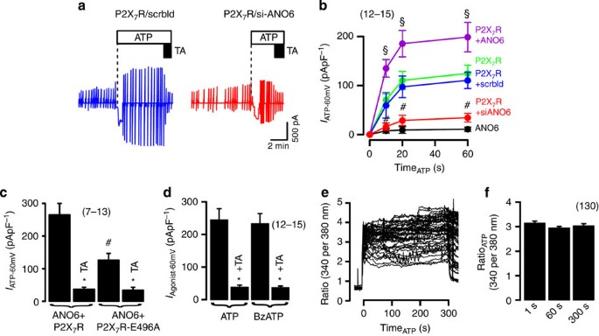Figure 2: ANO6 is activated through the stimulation of P2X7receptors. (a) Whole-cell currents activated by 3 mM ATP in HEK293 cells expressing P2X7R. Cells were treated with scrambled RNA (scrbld; left) or siRNA-ANO6 (si-ANO6; right). Cells were continuously voltage clamped between ±100 mV; ATP was applied at a holding voltage of −60 mV. TA (20 μM) was applied at the end of the recording to indicate activation of Cl−currents. (b) Time-dependent activation of whole-cell currents by ATP in HEK293 cells expressing P2X7R, ANO6 or both, and treated with scrbld RNA or siRNA-ANO6. (c) Effect of a point mutation in P2X7R on ATP - activated whole cell currents. (d) Summary of whole-cell currents activated by ATP (3 mM) or BzATP (100 μM), and inhibition of the activated current by TA (20 μM). (e) Original recordings demonstrating strong increase in free intracellular Ca2+concentrations (Fura-2; 340/380 nm) by ATP (3 mM) in cells coexpressing ANO6/P2X7R. (f) Summary of Fura-2 340/380 nm ratios indicating continuous high levels of cytosolic [Ca2+] during 300 s stimulation with ATP. Current data were obtained in fast whole-cell patch-clamp experiments. Mean±s.e.m.,n=number of cells.#§significant difference from P2X7R (P<0.05; analysis of variance). *significant inhibition by TA (P<0.05; pairedt-test). Figure 2: ANO6 is activated through the stimulation of P2X 7 receptors. ( a ) Whole-cell currents activated by 3 mM ATP in HEK293 cells expressing P2X 7 R. Cells were treated with scrambled RNA (scrbld; left) or siRNA-ANO6 (si-ANO6; right). Cells were continuously voltage clamped between ±100 mV; ATP was applied at a holding voltage of −60 mV. TA (20 μM) was applied at the end of the recording to indicate activation of Cl − currents. ( b ) Time-dependent activation of whole-cell currents by ATP in HEK293 cells expressing P2X 7 R, ANO6 or both, and treated with scrbld RNA or siRNA-ANO6. ( c ) Effect of a point mutation in P2X7R on ATP - activated whole cell currents. ( d ) Summary of whole-cell currents activated by ATP (3 mM) or BzATP (100 μM), and inhibition of the activated current by TA (20 μM). ( e ) Original recordings demonstrating strong increase in free intracellular Ca 2+ concentrations (Fura-2; 340/380 nm) by ATP (3 mM) in cells coexpressing ANO6/P2X 7 R. ( f ) Summary of Fura-2 340/380 nm ratios indicating continuous high levels of cytosolic [Ca 2+ ] during 300 s stimulation with ATP. Current data were obtained in fast whole-cell patch-clamp experiments. Mean±s.e.m., n =number of cells. #§ significant difference from P2X 7 R ( P <0.05; analysis of variance). *significant inhibition by TA ( P <0.05; paired t -test). Full size image Ano6 causes cellular effects downstream of P2X 7 receptors Phosphatidylserine (PS) exposure by stimulation of P2X 7 has been reported earlier [37] , and ANO6 was shown to operate as a Ca 2+ -dependent phospholipid scramblase [15] . We found that the activation of P2X 7 R induced exposure of PS to the outer membrane leaflet, when measured by annexin V binding. PS exposure was partially inhibited by TA but was abolished after siRNA knockdown of ANO6 expression ( Fig. 3a,b ). Stimulation of P2X 7 R by ATP-induced massive membrane blebbing, which was dependent on the function of ANO6 and the presence of functional P2X 7 R ( Fig. 3c,d ). Moreover, ATP-induced cell shrinkage preceding the membrane blebbing was detected by a transient fluorescence increase in calcein-loaded cells. Cell shrinkage leads to concentration of the calcein dye and thereby increases fluorescence, while cell swelling leads to decrease in fluorescence [22] . 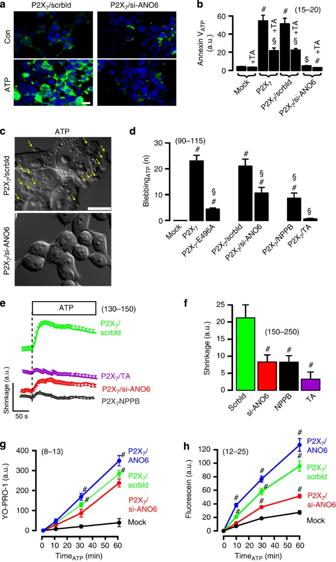Figure 3: ANO6 is part of the P2X7R pore conductance and responsible for cellular downstream effects. (a) ATP-induced annexin V binding in P2X7R-expressing HEK293 cells and effects of treatment with siRNA-ANO6 or scrambled RNA. Phospholipid scrambling and binding of annexin V (green fluorescence) was abolished after the knockdown of ANO6. (b) Summary of annexin V binding in mock-transfected and P2X7R-expressing HEK293 cells, and effects of the ANO6 blocker TA (10 μM). (c) Effect of ANO6 knockdown on ATP-induced membrane blebbing. Yellow arrows indicate multiple blebs in P2X7R-expressing HEK293 cells after application of ATP, which were absent after the knockdown of ANO6. (d) Effects of P2X7R-E496A mutation, ANO6 knockdown and ANO6 blockers NPPB (100 μM) and TA (20 μM) on ATP-induced membrane blebbing. (e,f) Effects of ANO6 knockdown and ANO6 blockers on ATP-induced cell shrinkage. (g) Effects of expression or siRNA knockdown of ANO6 and P2X7R on ATP-induced YO-PRO-1 uptake. YO-PRO-1 uptake was assessed by increase in fluorescence intensity. (h) Effects of expression or siRNA knockdown of ANO6 and P2X7R on ATP-induced fluorescein uptake. Mean±s.e.m.,n=number of cells and assays, respectively.#significant difference when compared with mock or scrambled (P<0.05; analysis of variance (ANOVA)).§significant inhibition by TA or various treatments (P<0.05; ANOVA). *significant inhibition by TA (P<0.05; pairedt-test). Scale bars, 20 μm. Figure 3: ANO6 is part of the P2X 7 R pore conductance and responsible for cellular downstream effects. ( a ) ATP-induced annexin V binding in P2X 7 R-expressing HEK293 cells and effects of treatment with siRNA-ANO6 or scrambled RNA. Phospholipid scrambling and binding of annexin V (green fluorescence) was abolished after the knockdown of ANO6. ( b ) Summary of annexin V binding in mock-transfected and P2X 7 R-expressing HEK293 cells, and effects of the ANO6 blocker TA (10 μM). ( c ) Effect of ANO6 knockdown on ATP-induced membrane blebbing. Yellow arrows indicate multiple blebs in P2X 7 R-expressing HEK293 cells after application of ATP, which were absent after the knockdown of ANO6. ( d ) Effects of P2X 7 R-E496A mutation, ANO6 knockdown and ANO6 blockers NPPB (100 μM) and TA (20 μM) on ATP-induced membrane blebbing. ( e , f ) Effects of ANO6 knockdown and ANO6 blockers on ATP-induced cell shrinkage. ( g ) Effects of expression or siRNA knockdown of ANO6 and P2X 7 R on ATP-induced YO-PRO-1 uptake. YO-PRO-1 uptake was assessed by increase in fluorescence intensity. ( h ) Effects of expression or siRNA knockdown of ANO6 and P2X 7 R on ATP-induced fluorescein uptake. Mean±s.e.m., n =number of cells and assays, respectively. # significant difference when compared with mock or scrambled ( P <0.05; analysis of variance (ANOVA)). § significant inhibition by TA or various treatments ( P <0.05; ANOVA). *significant inhibition by TA ( P <0.05; paired t -test). Scale bars, 20 μm. Full size image Subsequent to brief shrinkage, the cells appeared swollen and gradually lost their calcein signal, a phenomenon that had been observed earlier in lymphocytes [31] . Initial shrinkage relied on the presence and function of ANO6 ( Fig. 3e,f ). These data demonstrate that ANO6 is central to the deleterious cellular effects downstream of P2X 7 R. Similar effects of ANO6 on cellular volume have been observed earlier [38] and are described below for macrophages ( Fig. 4f,g , Supplementary Fig. 6e,f ). 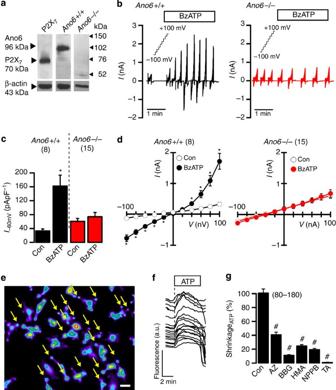Figure 4: Stimulation of P2X7R in macrophages activates Ano6 and changes cell volume. (a) Western blot demonstrating the expression of P2X7R and Ano6 in mouseAno6+/+and lack of expression of Ano6 inAno6−/− macrophages. (b) Activation of whole-cell currents by 100 μM BzATP in macrophages fromAno6+/+mice and lack of activation in macrophages fromAno6−/− mice. (c) Summary of current densities measured in wt andAno6-KOmacrophages. (d) Current/voltage relationships of ATP-induced whole-cell currents from wt andAno6-KOmacrophages. (e) Membrane blebbing in mouse macrophages exposed to 3 mM ATP. Macrophages have been loaded with calcein. (f) Initial shrinkage and subsequent swelling with loss of fluorescence inAno6+/+macrophages exposed to ATP. Volume changes were assessed by change in calcein fluorescence. (g) ATP-induced initial shrinkage (%) and attenuation of shrinkage by inhibition of P2X7R (100 nM AZ11645373; 10 μM Brilliant blue G; 40 μM 5-(N,N-hexamethylene)amiloride) or blocking of Ano6 (100 μM NPPB, 10 μM TA). Mean±s.e.m.,n=number of cells.#significant difference when compared with control (P<0.05; analysis of variance). *significant activation by BzATP (P<0.05; pairedt-test). Scale bar, 20 μm. Figure 4: Stimulation of P2X 7 R in macrophages activates Ano6 and changes cell volume. ( a ) Western blot demonstrating the expression of P2X 7 R and Ano6 in mouse Ano6+/+ and lack of expression of Ano6 in Ano6 −/− macrophages. ( b ) Activation of whole-cell currents by 100 μM BzATP in macrophages from Ano6+/+ mice and lack of activation in macrophages from Ano6 −/− mice. ( c ) Summary of current densities measured in wt and Ano6-KO macrophages. ( d ) Current/voltage relationships of ATP-induced whole-cell currents from wt and Ano6-KO macrophages. ( e ) Membrane blebbing in mouse macrophages exposed to 3 mM ATP. Macrophages have been loaded with calcein. ( f ) Initial shrinkage and subsequent swelling with loss of fluorescence in Ano6+/+ macrophages exposed to ATP. Volume changes were assessed by change in calcein fluorescence. ( g ) ATP-induced initial shrinkage (%) and attenuation of shrinkage by inhibition of P2X 7 R (100 nM AZ11645373; 10 μM Brilliant blue G; 40 μM 5-( N , N -hexamethylene)amiloride) or blocking of Ano6 (100 μM NPPB, 10 μM TA). Mean±s.e.m., n =number of cells. # significant difference when compared with control ( P <0.05; analysis of variance). *significant activation by BzATP ( P <0.05; paired t -test). Scale bar, 20 μm. Full size image Pore formation is ANO6 dependent Numerous reports demonstrate the formation of a large pore conductance by the activation of P2X 7 R that is permeable for fluorescent dyes such as YO-PRO-1, fluorescein or calcein [7] , [8] , [39] , [40] . We therefore analysed whether ANO6 also contributes to P2X 7 R pore formation. In the absence of P2X 7 R (mock), ATP or the Ca 2+ ionophore A23187 was unable to induce the uptake of YO-PRO-1 into HEK293 ( Fig. 3g , Supplementary Fig. 3c,d ). In contrast, YO-PRO-1 uptake were detected after ATP stimulation of P2X 7 R-overexpressing cells, which was only slightly attenuated by knockdown of ANO6 ( Fig. 3g ), but strongly inhibited by blockers of ANO6 such as NPPB and TA ( Supplementary Fig. 3f ). Blockers of P2X 7 R (HMA, AZ) and mutations within P2X 7 R (P2X 7 -E496A or P2X 7 -436X) also inhibited YO-PRO-1 uptake ( Supplementary Fig. 3e,f ). YO-PRO-1 uptake was relatively slow in HEK293 cells probably due to low rate (40%) of transfection of P2X 7 R or low endogenous levels of ANO6. We therefore measured ATP-induced YO-PRO-1 uptake also in single human THP-1 macrophages. YO-PRO-1 uptake was strongly inhibited by siRNA knockdown of ANO6 by two different siRNAs ( Supplementary Fig. 6c,d ). Moreover, uptake of the negatively charged dye fluorescein was inhibited by siRNA knockdown of endogenous ANO6, but was augmented by overexpression of exogenous ANO6, respectively ( Fig. 3h ). This suggests that both P2X 7 R containing an intact C terminus, as well as ANO6, are required for dye uptake and large conductance induced by ATP. P2X 7 activates Ano6 in macrophages Macrophages express high levels of P2X 7 R ( Supplementary Fig. 6a,c ). Numerous studies report a role of P2X 7 R during inflammation, immune defense and host–pathogen response (for review see refs 1 , 27 ). We detected the expression of both mRNA and protein of P2X 7 R and Ano6 in mouse and human macrophages using RT–PCR and western blotting ( Fig. 4a , Supplementary Figs 5a,6a,c ). Large whole-cell currents were activated in Ano6-expressing wt macrophages by either ATP or BzATP, and the activation was inhibited by TA ( Fig. 4b–d , Supplementary Fig. 5b–e ). In contrast, no whole-cell currents were activated by BzATP in macrophages of Ano6 −/− mice, apart from a small negative current ( Fig. 4b–d ). This result indicates an essential contribution of Ano6 to P2X 7 R-induced whole-cell currents in macrophages. Interestingly, when Ano6 −/− macrophages were stimulated with ATP (3 mM) instead of BzATP, an inward current (Δ I −100 mV =169±28 pA/pF; n =5) was activated, similar to that obtained in Ano6+/+ animals (Δ I −100 mV =189±36 pA/pF; n =4). Thus, additional purinergic receptors in macrophages (P2X 4 , P2Y 2 ) may be stimulated by ATP, leading to activation of other anoctamins such as Ano1, or coupling of Ano6/P2X 7 may not be mandatory for stimulation by ATP. Ano6+/+ macrophages demonstrated pronounced membrane blebbing when exposed to ATP ( Fig. 4e , Supplementary Fig. 7 ). Blebbing followed brief cell shrinkage (measured as increase in calcein fluorescence) and loss of calcein fluorescence ensued blebbing. Shrinkage and loss of fluorescence were inhibited by blockers of P2X 7 R (Brilliant blue G, HMA, AZ116453739) and inhibitors of Ano6 (NPPB and TA; Fig. 4g ). In macrophages from two Ano6 −/− animals, we did not observe ATP-induced cell shrinkage or cell rupture. Moreover, ANO6 knockdown in human THP-1 macrophages significantly reduced ATP-induced shrinkage ( Supplementary Fig. 6e,f ). This suggests that ATP-induced volume changes in macrophages and membrane blebbing is ANO6 dependent. Changes in cell volume are intimately related to the ability of cells to migrate, which is also an important function of macrophages [41] , [42] . Monocyte chemoattractant protein-1 (MCP-1) is one of the key chemokines that regulate migration and infiltration of macrophages and other immune cells [43] . Notably, a role of anoctamins for cell migration has been identified earlier [44] , [45] . We found that in mouse macrophages, MCP-1-induced migration through Boyden chambers was inhibited by the Ano6 blocker TA, suggesting a role of Ano6 for migration of mouse macrophages ( Supplementary Fig. 6a,b ). More importantly, MCP-1-induced migration was absent in macrophages from Ano6 −/− animals, and inhibition of migration by TA was abolished ( Supplementary Fig. 6b ). While the expression of Ano6 was absent in Ano6 −/− macrophages, the expression of P2X 7 R remained unchanged ( Supplementary Fig. 6a ). We further confirmed the role of ANO6 for migration by downregulation of Ano6 expression in human THP-1 macrophages using two different siRNAs: ANO6 knockdown abolished the effects of MCP-1 and TA ( Supplementary Fig. 6c,g ). Activation of Ano6 is essential for macrophage function We examined whether the activation of Ano6 is essential for further cellular effects downstream of P2X 7 R. Apoptosis is one of the key events that take place after the stimulation of P2X 7 R. In vivo macrophages may be exposed to high extracellular ATP probably only for short periods of time, during tissue damage or inflammation [42] . We therefore exposed mouse peritoneal macrophages to 3 mM ATP for only 5 min, and measured activation of caspase-3 during the following 12 h. ATP was applied without previous priming by lipopolysaccharide, which exerted an immediate proapoptotic effect ( Supplementary Fig. 8a ). Transient exposure to ATP induced delayed activation of caspase-3, which was completely suppressed by TA ( Fig. 5a,b , Supplementary Fig. 8c,d ). Moreover, the activation of caspase-3 was significantly reduced in macrophages from Ano6 null mice ( Fig. 5c ) or after the knockdown of Ano6 expression in macrophages from wt animals ( Supplementary Fig. 8b,c ). 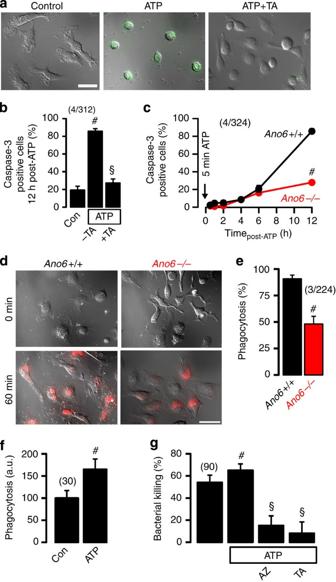Figure 5: Effects of P2X7R on macrophage functions are controlled by Ano6. (a) Activation of caspase-3 in mouse macrophages by 3 mM ATP and inhibition by 20 μM TA. (b) Percentage of caspase-3-positive cells 12 h after exposure (5 min) to 3 mM ATP and inhibition by TA. (c) Time course for caspase-3-positive macrophages from wt andAno6−/− animals. (d) Phagocytosis (1 h) of fluorescent bioparticles by macrophages from wt andAno6−/− animals. (e) Percentage of phagocytosis-positivewtandAno6−/− macrophages after 1 h exposure to bioparticles. (f) Fluorescence intensity after 1 h of phagocytosis and effects of initial 5 min exposure to 3 mM ATP. (g) Effect of initial exposure to 3 mM ATP on bacterial killing, and inhibition of killing by 100 nM AZ11645373 and 20 μM TA. Mean±s.e.m.,n=number of cells and assays, respectively.#significant difference when compared with control or toAno6+/+(P<0.05; analysis of variance (ANOVA)).§significant inhibition by blockers (P<0.05; ANOVA). Scale bars, 20 μm. Figure 5: Effects of P2X 7 R on macrophage functions are controlled by Ano6. ( a ) Activation of caspase-3 in mouse macrophages by 3 mM ATP and inhibition by 20 μM TA. ( b ) Percentage of caspase-3-positive cells 12 h after exposure (5 min) to 3 mM ATP and inhibition by TA. ( c ) Time course for caspase-3-positive macrophages from wt and Ano6 −/− animals. ( d ) Phagocytosis (1 h) of fluorescent bioparticles by macrophages from wt and Ano6 −/− animals. ( e ) Percentage of phagocytosis-positive wt and Ano6 −/− macrophages after 1 h exposure to bioparticles. ( f ) Fluorescence intensity after 1 h of phagocytosis and effects of initial 5 min exposure to 3 mM ATP. ( g ) Effect of initial exposure to 3 mM ATP on bacterial killing, and inhibition of killing by 100 nM AZ11645373 and 20 μM TA. Mean±s.e.m., n =number of cells and assays, respectively. # significant difference when compared with control or to Ano6+/+ ( P <0.05; analysis of variance (ANOVA)). § significant inhibition by blockers ( P <0.05; ANOVA). Scale bars, 20 μm. Full size image Mouse macrophages showed strong spontaneous phagocytic activity even without the addition of ATP, as demonstrated by phagocytosis of fluorescence-conjugated bioparticles ( Fig. 5d , Supplementary Fig. 8e,f ). All cells showed phagocytosed bioparticles after 60 min of exposure, as indicated by visual red fluorescence. However, phagocytosis was significantly inhibited by NPPB and TA ( Supplementary Fig.8f ). The amount of phagocytosis (as measured by fluorescence intensity) was further augmented by short term application (5 min) of ATP ( Fig. 5f ). Notably macrophages from Ano6 −/− mice demonstrated reduced spontaneous phagocytosis, when compared with wt animals ( Fig. 5d,e ). We finally tested in an E. coli viability assay the ability of macrophages to destroy phagocytosed bacteria. Bacterial killing by macrophages was observed without additional ATP, but was further enhanced by short ATP-exposure. In contrast, killing was largely inhibited by AZ and TA ( Fig. 5g ). This result suggests a release of ATP by bacterial contact, as demonstrated previously [46] . Released ATP binds to purinergic receptors thereby allowing chemotactic navigation via P2Y 2 and P2Y 12 (ref. 42 ). Macrophage responses to bacterial infection are augmented via P2X 7 R signalling, as shown here and in an earlier study [10] , leading to augmented bacterial killing [47] , [48] . Taken together, the present data suggest a crucial role of Ano6 for the cellular effects downstream of P2X 7 R, and for the innate immunity function of macrophages ( Fig. 6 ). 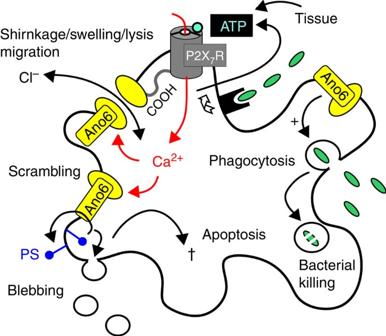Figure 6: Model for the role of ANO6 in macrophages. Lectin-type binding of bacteria to the macrophage membrane induces ATP release by unknown mechanisms. Autocrine ATP binding activates P2X7R, increases intracellular Ca2+and activates Cl−currents, leading to immediate cell shrinkage. Ano6 induces phospholipid scrambling, which leads to subsequent plasma membrane blebbing and apoptosis. Activation of Ano6 whole-cell currents also supports the migration of macrophages, thereby enhancing the chance for phagocytosis and subsequent killing of phagocytosed bacteria. Figure 6: Model for the role of ANO6 in macrophages. Lectin-type binding of bacteria to the macrophage membrane induces ATP release by unknown mechanisms. Autocrine ATP binding activates P2X 7 R, increases intracellular Ca 2+ and activates Cl − currents, leading to immediate cell shrinkage. Ano6 induces phospholipid scrambling, which leads to subsequent plasma membrane blebbing and apoptosis. Activation of Ano6 whole-cell currents also supports the migration of macrophages, thereby enhancing the chance for phagocytosis and subsequent killing of phagocytosed bacteria. Full size image The present results show that opening of P2X 7 R channels causes immediate influx of Ca 2+ that activates a large whole-cell current with a delay of only seconds to 2 min, depending on the cell type. This whole-cell conductance allows permeation of the fluorescent molecules YO-PRO-1, fluorescein and calcein and thus relates to the large P2X 7 R ‘pore’ conductance [5] , [39] , [40] , [49] . Whether P2X 7 R channels dilate to a dye-permeable pore on continuous binding of ATP [50] , [51] or whether dyes use one or several independent permeation pathways [7] , [8] , [9] , [39] , [40] , is still a matter of debate. These pathways may be activated through increase in intracellular Ca 2+ and/or via a signalling complex located at the C terminus of P2X 7 R. In either event, the present data show that ANO6 (i) is activated by the P2X 7 R-mediated increase in intracellular Ca 2+ and (ii) is in part responsible for delayed pore conductance and dye uptake. Previous work [17] , [18] , [19] , [20] and present results indicate that ANO6 requires high intracellular [Ca 2+ ] i to be activated, corresponding to the high [Ca 2+ ] i levels provided by activation of P2X 7 R. Moreover, recent data from mouse and human ANO6 and the reconstituted ANO6 homologue from Aspergillus fumigatus suggest a rather large pore size for ANO6 (refs 16 , 18 , 21 ). Because we could coimmunoprecipitate ANO6 and P2X 7 R, we speculate that ANO6 is part of a macromolecular complex containing P2X 7 R and possibly different diffusion pathways for cations and anions [4] , [7] . In this regard, the unique extended C terminus of P2X 7 R appears essential for pore formation and subsequent cell death, as suggested earlier [49] , [52] . We show that ANO6 participates in many of the essential cellular responses downstream of P2X 7 R like (i) Initial cell shrinkage, (ii) membrane blebbing, (iii) membrane phospholipid scrambling and (iv) apoptosis ( Fig. 6 ). These findings support the general concept of cell shrinkage being an early and essential step, triggering the cell death machinery [53] . Notably, evidence for cell shrinkage due to activation of ANO6 has been shown previously, and ANO6 currents were activated by proapoptotic stimuli [17] , [22] , [24] , [38] . Sequential shrinkage/swelling and translocation of PS on P2X 7 R-stimulation have also been reported for lymphocytes [31] . Our own data indicate that the stimulation of P2X 7 R activates ANO6 in Xenopus oocytes, HEK293 cells, macrophages and Jurkat T lymphocytes ( Supplementary Fig. 9 ). The importance of Cl − ions for P2X 7 R-induced cell shrinkage and subsequent cell death has been also suggested in previous studies [35] , [54] . ANO6 does not produce classical volume-regulated Cl − currents ( I Cl, swell ) with typical time-dependent inactivation [55] . It is nevertheless activated by apoptotic stimuli and cell swelling, and thus forms the Ca 2+ -dependent component of volume-regulated Cl − currents [22] , [24] , [38] . Phospholipid scrambling induced by the stimulation of P2X 7 R is probably due to strong [Ca 2+ ] i increase, inducing the scramblase activity of ANO6 (refs 15 , 17 ), and may also support membrane blebbing, two intimately related cellular events [53] , [56] . Activation of ANO6 by stimulation of P2X 7 R affects essential macrophage functions such as (i) migration, (ii) phagocytosis of bacteria and (iii) bacterial killing ( Fig. 6 ). Autocrine purinergic signalling has been shown recently to control chemotaxis and migration of macrophages [42] . Both ANO1 and ANO6 contribute to migration also in other cell types, which has large implications for tumour metastasis [41] , [44] , [45] , [57] . The present report now establishes a role of ANO6 for migration of macrophages, which has an impact on phagocytic activity and subsequent bacterial killing. In situ macrophages are probably only transiently exposed to high extracellular ATP concentrations [10] , [42] . The present data show that only 5 min exposure to 3 mM ATP enhances phagocytosis and bacterial killing, and induces delayed apoptosis, corresponding to the delayed ATP-induced apoptosis observed in an earlier report [10] . A role of P2X 7 R signalling in macrophages for killing of mycobacteria [47] , [58] and other pathogens [27] has been demonstrated earlier. We may speculate that P2X 7 R-induced phagolysosomal fusion [27] , [59] is supported by ANO6 after engulfment of bacteria. Notably, Ano1 was shown recently to support endosomal acidification and renal tubular protein reabsorption [60] . Taken together, we demonstrate that ANO6 is central to cellular effects downstream of the P2X 7 receptor. It therefore reflects a potential pharmacological target to interfere with immunological processes and cellular apoptosis. Anoctamin 6-knockout mice Generation of Anoctamin 6 (TMEM16F) knockout mice (C57Bl6, 6–12 weeks, male or female) has been described earlier [28] . These mice were kindly provided by Professor Dr A. Vortkamp (Department of Developmental Biology, University of Essen, Germany). Procedures were performed in compliance with the guidelines for the welfare of experimental animals issued by the Federal Government of Germany, and were approved by the local board. Cell culture and cDNA Human embryonic kidney (HEK293; ATCC) cells were grown in Dulbecco’s modified Eagle’s medium supplemented with 10% fetal bovine serum. Cells were incubated in 5% CO 2 at 37 °C. The vectors pcDNA3.1-hP2X7, the oocyte expression vectors pNKS4-hP2X7-C-terminal truncated (436aa), pNKS4-hP2X7 and pNKS4-hP2X7-His tagged were kindly provided by Professor Schmalzing and Michaela Stoll (Inst. für Pharmakologie & Toxikologie, Universitätsklinikum der RWTH Aachen, Germany). The vectors pcDNA3.1-hP2X7/E496A and pNKS4-hP2X7/E496A-His were produced by PCR-based site-directed mutagenesis. pcDNA3.1-hP2X7-C-terminal truncated and pcDNA3.1-cmyc/hP2X7 were generated by subcloning using PCR techniques. Human ANO6 cDNA was amplified from total RNA of 16HBE cells by RT–PCR. All sequences were verified by sequencing. The expression of human ANO6 was suppressed by two to three sets of siRNA. Duplexes of 25 nucleotides of Stealth RNAi siRNA were designed and synthesized by Invitrogen ( Supplementary Table 2 ). Plasmids or siRNA were transfected into HEK293 cells using standard methods (Lipofectamine, Invitrogen). Cells were examined 48 or 72 h after transfection. Patch clamp Cells grown on coverslips were mounted in a perfused bath on the stage of an inverted microscope (IM35, Zeiss) and kept at 37 °C. The bath was perfused continuously with Ringer solution (mM: NaCl 145, KH 2 PO 4 0.4, K 2 HPO 4 1.6, D -glucose 6, MgCl 2 1, Ca-gluconate 1.3, pH 7.4) at about 10 ml min −1 . Patch-clamp experiments were performed in the fast whole-cell configuration. Patch pipettes had an input resistance of 3–4 MΩ, when filled with an intracellular like solution containing (mM) KCl 30, K-gluconate 95, NaH 2 PO 4 1.2, Na 2 HPO 4 4.8, EGTA 1, Ca-gluconate 0.758, MgCl 2 1.034, D-glucose 5, ATP 3. pH was 7.2, the Ca 2+ activity was 0.1 μM. The access conductance was measured continuously and was 90–140 nS (EPC 9 amplifier, List Medical Electronics, Darmstadt, Germany). In regular intervals, membrane voltages ( V c ) were clamped in steps of 20 mV from −100 to +100 mV and the membrane conductance G m was calculated from the measured current ( I ) and V c values according to the Ohm’s law. Two-electrode voltage clamp Oocytes were harvested from Xenopus laevis according to the German regulations governing animal experiments. Oocytes were defolliculated for 1 h at 18 °C with 1.5 mg ml −1 collagenase type V (Sigma) in OR2 solution (in mmol l −1 ): 82.5 NaCl, 2 KCl, 1 MgCl 2 and 5 HEPES pH 7.55. Oocytes were injected with 10 ng (47 nl double-distilled water) of cRNA encoding P2X7, P2X7-E496 or P2X7-C-terminal truncated. cRNA was transcribed in vitro after linearization, using the appropriate promoter and RNA-polymerase (T3, T7 or SP6). Oocytes were maintained in ND97 solution (in mmol l −1 ): 96 NaCl, 2 KCl, 1.8 CaCl 2 , 1 MgCl 2 , 5 HEPES, 2.5 Na-pyruvate, 0.5 theophylline and 0.01 mg ml −1 gentamycin, pH 7.55 at 18 °C. Two to four days after injection, membrane currents were measured by impaling two electrodes (Harvard Apparatus, UK) filled with 3 mol l −1 KCl, which had a resistance of less than 1 MΩ. The bath was continuously perfused at a rate of 5 ml min −1 with ND96 solution (in mmol/l): 96 NaCl, 2 KCl, 1.8 CaCl 2 , 1 MgCl 2 , 5 HEPES and 2.5 Na-pyruvate, pH 7.55. The voltage drop across the serial resistance was optimized to zero using two bath electrodes and a virtual ground head stage. Oocytes were continuously voltage clamped between −60 and +40 mV (oocyte clamp amplifier, Warner Instruments, USA) in steps of 10 mV, each 1 s. All experiments were conducted at room temperature. Reverse transcriptase PCR and real-time PCR Total RNA was isolated from human B lymphocytes, macrophages or from Xenopus laevis oocytes using RNeasy Mini-Kit (Qiagen; Hilden, Germany). Two μg of total RNA was reverse transcribed in 50 μl for 1 h at 40 °C using random primer and reverse transcriptase (RT). Thirty cycles of RT–PCR was performed using standard procedures (GoTaq DNA Polymerase, Promega), 1 μl RT and primers for P2X7 and anoctamins (0.5 μM, Supplementary Table 1 ). For semi-quantitative comparison, glyceraldehyde 3-phosphate dehydrogenase was amplified. Products were analysed on ethidium bromide-stained 2% agarose gels. The real-time PCR was performed in 10 μl of mixture (5 μl of 2 × SYBR Green I master mix, 0.5 μM of each forward and reverse primer (LightCycler, Roche, Germany) ( Supplementary Table 1 ). The cycle threshold value was accessed by LightCycler 480 Software. The cycle threshold values of the human ANO6 and β-actin mRNAs were calculated from the equations and standard curves. Samples were analysed in triplicate of each and human ANO6 levels were normalized to the corresponding β-actin. Western blotting Protein was isolated from transfected HEK293 cells using lysis buffer (50 mM Tris, 150 mM NaCl, 1 mM EDTA, 1% NP-40, 100 mM dithiothreitol and 1% proteinase inhibitor cocktail) and protein concentration was measured by Bradford. Samples were run on SDS–polyacrylamide gel electrophoresis gel and transferred to polyvinylidene difluoride membrane (GE Healthcare Europe, Germany) using wet transfer (BioRad, Germany). Membranes were incubated with 1:1,000 anti-GFP rabbit antibody (# A11122; Invitrogen, Germany), 1:500 rabbit anti-ANO6 antibody (ARP44761; Aviva System Bio, USA), 1:500 rabbit anti-P2X7 antibody (APR-008; Alomone Labs, Israel) and 1:500 mouse anti-ß-actin antibody (sc-47778; Santa Cruz, Germany) overnight at 4 °C. Proteins were visualized using anti-rabbit horseradish peroxidase-conjugated antibody (Acris, Germany) or anti-mouse horseradish peroxidase-conjugated antibody (Santa Cruz, Germany) and chemiluminescent substrate (Pierce, Thermo Scientific). For detection of expression of anoctamin 6 and P2X 7 , macrophages were collected as described below. After isolation of protein and separation on SDS–polyacrylamide gel electrophoresis, proteins were detected using 1:500 rabbit anti-ANO6 (ARP44761; Aviva System Bio, USA) and 1:500 rabbit anti-P2X7 antibody (APR-008; Alomone Labs, Israel). Images have been cropped for presentation. Full size images are presented in Supplementary Figs 10–12 . Immunocytochemistry Transfected HEK293 cells were grown on glass coverslips and fixed for 10 min with 4% (w/v) paraformaldehyde at room temperature. Cells were incubated for 5 min with 0.1% SDS in PBS. After washing, the cells were permeabilized and blocked with 2% (w/v, PBS) bovine serum albumin and 0.04% (v/v, PBS) Triton-X-100 and incubated for 1 h with primary anti-P2X7 rabbit antibody (1:500) at 37 °C. Binding of the primary antibody was visualized by incubation with a secondary antibody conjugated with Alexa 568. Green GFP fluorescence was used to indicate ANO6-GFP expression. Nuclei were stained with Hoe33342 (0.1 μg ml −1 PBS, Aplichem, Darmstadt, Germany). Cells were mounted on glass slides with fluorescent mounting medium (DAKO Cytomation, Hamburg, Germany) and examined with an ApoTome Axiovert 200 M fluorescence microscope (Zeiss, Göttingen, Germany). Annexin V binding and dye uptake assays HEK293 cells grown on glass coverslips were treated with ATP with or without TA (TA; 10 μM). After 5 min, the cells were incubated with annexin V-FITC (BD Pharmingen, Germany) for 15 min at 20 °C. Cells were subsequently analysed using ApoTome Axiovert 200M fluorescence microscope (Zeiss, Germany) and SlideBook Digital Microscopy Software (Corolado, USA). Membrane permeabilization observed during apoptosis was assayed using the positively charged carbocyanine nucleic acid dye YO-Pro-1 (Life Technologies). Cells grown and transfected in 96-well plates were washed and resuspended in ringer solution. YO-Pro-1 was added at a final concentration of 1 μM. Cells were incubated with 3 mM ATP with and without the P2X 7 -inhibitors AZ11645373 (25 nM) and 5-( N , N -hexamethylene)amiloride (40 μM), or the anoctamin Cl − channel inhibitors NPPB (100 μM NPPB), NFA (10 μM) or AO1 (20 μM). YO-Pro-1 fluorescence (excitation 480 nm/emission 520 nm) was measured every minute for 3 h at 37 °C using the plate reader NOVOstar (BMG LABTECH, Germany). HEK293 cells grown in 96-well plates were treated with 3 mM ATP for 6 h at 37 °C in the presence and absence of TA. Luminogenic caspase-3/7 substrate (Promega, Germany) was added into each well and mixed at room temperature. The luminescence was measured using the plate reader NOVOstar (BMG LABTECH, Germany). Apoptosis in primary peritoneal macrophages was assessed by NucView 488 Caspase-3 assay kit (Biotum, Germany). In brief, macrophages were incubated with DEVD-NucView488 substrate and apoptotic cells were analysed using the plate reader NOVOstar before and after treatment with 3 mM ATP. Photos were taken by an Axiovert 200M fluorescence microscope with ApoTome (Zeiss, Germany). Intracellular Ca 2+ concentrations and cell volume changes HEK293 cells were seeded on glass coverslips and loaded with 2 μM Fura-2/AM and 0.02% Pluronic F-127 (Life Technologies, Germany) in ringer solution (mmol l −1 : NaCl 145; KH 2 PO 4 0,4; K 2 HPO 4 1,6; Glucose 5; MgCl 2 1; Ca 2+ -Gluconat 1,3) for 1 h at room temperature. Fluorescence was detected in cells perfused with Ringer’s solution at 37 °C using an inverted microscope (Axiovert S100, Zeiss, Germany) and a high-speed polychromator system (VisiChrome, Germany). Fura-2 was excited at 340/380 nm, and emission was recorded between 470 and 550 nm using a CoolSnap camera (CoolSnap HQ, Visitron). For volume measurements, macrophages were cultured on glass covers for 2 days and loaded with 1 μM calcein-AM (Life Technologies, Germany) and 0.01% Pluronic F-127 (Life Technologies, Germany) in ringer solution for 1 h at room temperature. Calcein was excited at 490 nm, and the emission was recorded between 520 and 550 nm. Control of experiment, imaging acquisition and data analysis were done with the software package Meta-Fluor (Universal imaging, USA) and Origin (OriginLab Corporation, USA). Isolation and culture of primary peritoneal macrophages Mice were anaesthetized using CO 2 and killed via cervical delocation. Intraperitoneal lavage was performed by delivering 10 ml of cold PBS into the abdomen with a 19-gauge needle. The cells were collected with a 24-gauge needle, plated in 12-well plates (500 μl per well) and incubated at 37 °C. After 1 h, the non-adherent cells were removed by washing five times with PBS. The adherent cells were cultured in RPMI media supplemented with 10% fetal bovine serum, 1% PS and Glutamine 200 nM in 5% CO 2 at 37 °C (Life Technologies, Germany). Phagocytosis assay Macrophages were seeded on 18-mm glass coverslips. After 5 min incubation with 3 mM ATP, the cells were incubated with the inhibitors TA (10 μM) or AZ11645373 (50 nM) in RPMI media for 5 h. To measure phagocytosis, the macrophages were incubated with 0.4 mg pHrodo E. coli bioparticles conjugate (Life Technologies, Germany) in 1 ml ringer solution for 1 h at 37 °C. After washing, cellular fluorescence was measured using an ApoTome Axiovert 200 M fluorescence microscope and the software AxioVision (Zeiss, Germany). To calibrate the fluorescence intensity to pH, cells were incubated in MES buffer at pH 7.5 and 4 in the presence of 5 μM nigericin. E. coli viability assay Macrophages were infected with E. coli XL1 Blue MRF´ (Agilent Technologies) for 1 h at 37 °C. After 5 min incubation with 3 mM ATP, cells were incubated with the inhibitors TA (10 μM) or AZ11645373 (50 nM) in ringer solution for 0, 3 and 6 h. After washing, the cells were lysed in Luria-Bertani media with 0.4% saponin at 37 °C for 2 h. The number of viable E. coli was accessed by determination of colony-forming units on tetracycline-containing agar plates. Boyden chamber assay Migration of macrophages was measured using the Cell Biolabs CytoSelect 96-well Cell Migration Assay Kit (Cell Biolabs, USA). In brief, the macrophages were seeded on polycarbonate membrane with 5 μm pore size for 1 h. Medium of the upper chamber was replaced by serum-free RPMI medium containing TA (10 μM), AZ11645373 (50 nM), 100 μM NPPB, 10 μM NFA or 20 μM AO1. To the lower chamber, RPMI with MCP-1 (10 nM) as the chemoattractant was added. After 4 h incubation at 37 °C, migrated macrophages were lysed and incubated with CyQuant GR dye solution at 20 °C for 20 min. Fluorescence (excitation 480 nm/emission 520 nm) was measured using the plate reader NOVOstar (BMG LABTECH, Germany). Materials and statistical analysis All animal experiments were approved by local authorities and were conducted according to the guidelines of the American Physiological Society and the German law for welfare of animals. All compounds used were of highest available grade of purity and were from Sigma or Merck. All cell culture reagents were from Invitrogen. Experiments were repeated 4–30 times, exact numbers are reported in the figures. Data are reported as mean±s.e.m. Student’s t -test (for paired or unpaired samples as appropriate), Fisher’s exact tests and analysis of variance were used for statistical analysis. P <0.05 was accepted as significant difference. How to cite this article : Ousingsawat, J. et al . Anoctamin 6 mediates effects essential for innate immunity downstream of P2X 7 receptors in macrophages. Nat. Commun. 6:6245 doi: 10.1038/ncomms7245 (2015).